Repeated growth and bubbling transfer of graphene with millimetre-size single-crystal grains using platinum Large single-crystal graphene is highly desired and important for the applications of graphene in electronics, as grain boundaries between graphene grains markedly degrade its quality and properties. Here we report the growth of millimetre-sized hexagonal single-crystal graphene and graphene films joined from such grains on Pt by ambient-pressure chemical vapour deposition. We report a bubbling method to transfer these single graphene grains and graphene films to arbitrary substrate, which is nondestructive not only to graphene, but also to the Pt substrates. The Pt substrates can be repeatedly used for graphene growth. The graphene shows high crystal quality with the reported lowest wrinkle height of 0.8 nm and a carrier mobility of greater than 7,100 cm 2 V −1 s −1 under ambient conditions. The repeatable growth of graphene with large single-crystal grains on Pt and its nondestructive transfer may enable various applications. Graphene, a two-dimensional honeycomb lattice of sp 2 -bonded carbon atoms, has attracted worldwide interest since its experimental isolation from graphite [1] . The extremely high intrinsic carrier mobility [2] , high transparency [3] and remarkable tensile strength [4] make graphene a promising material in a wide range of applications, including electronics, spintronics, optoelectronics, sensors, batteries and supercapacitors [2] , [5] . Monolayer and few-layer graphene with high crystal quality have been prepared by micromechanical cleavage from graphite [1] , thermal decomposition of SiC [6] and epitaxial or chemical vapour deposition (CVD) growth on metals such as Ru [7] , [8] , Pt [9] , Ni [10] , [11] , [12] and Cu [13] , [14] , [15] , [16] , [17] , [18] , [19] , [20] . In particular, CVD growth on Cu foils has recently attracted increasing attention, because of its great potential for the growth of large-area monolayer graphene [13] , [14] , [15] , [16] , [19] , [20] . There is increasing evidence of the polycrystalline nature of graphene prepared by various growth methods [6] , [16] , [17] , [18] , [19] , [21] , [22] , [23] . Thermal decomposition of SiC yields graphene with a grain size of tens of micrometres [6] . Graphene films grown on Cu by CVD are formed from grains smaller than 10 μm (refs 16 , 17 , 18 , 21 ), even on single-crystal Cu(111) [17] . Recently, individual hexagonal graphene grains have been prepared on Cu foils by ambient pressure CVD (AP-CVD), but show a small size up to 20 μm (ref. 22 ). Graphene grains of hundreds of micrometres in size were grown on Cu foils using low pressure CVD (LP-CVD), but they resembled dendrites and had a high edge roughness [19] . Single-crystal Ru [7] , [8] and Ni [12] have also been demonstrated to be able to grow large graphene grains up to millimetre size in ultra-high vacuum. However, it remains a great challenge to transfer graphene from these single-crystal metals to other substrates. The currently used transfer processes are mostly based on the complete etching of metal substrates in suitable etchants [10] , [11] , [12] , [13] , [14] , [15] , [16] , [20] , which not only leads to inevitable damage to the graphene, the production of metal residues and serious environmental pollution, but also increases production cost. In particular, these processes are not suitable for the transfer of graphene from chemically inert or noble metal substrates, because these metals are difficult to etch away completely or have a high cost. The graphene grown on such substrates was mainly studied using surface techniques without transfer to other substrates [24] , which limits its study and applications to some extent. Very recently, an electrochemical delamination method was reported to transfer graphene grown on Cu to another substrate [25] . During this transfer process, the Cu substrate was also partially etching, with about 40 nm of Cu in thickness being etched away for each transfer, and can be only used for hundreds of growth and transfer processes. Here we report the growth of millimetre-size, single-crystal hexagonal graphene grains and graphene films joined from such grains on Pt substrates by AP-CVD, and a bubbling method to transfer these graphene grains and graphene films from Pt onto arbitrary substrates. This bubbling method is nondestructive, not only to the graphene but also to the Pt substrates, which allows for the repeated growth of graphene on Pt. The Pt substrates can be repeatedly used with almost no limit, and the graphene obtained on a repeatedly used Pt substrate has almost the same quality as that obtained originally. The graphene shows a high crystalline quality with the lowest wrinkle height reported until now and a carrier mobility of greater than 7,100 cm 2 V −1 s −1 . Growth of single-crystal graphene grains and continuous films Large hexagonal single-crystal graphene grains, and graphene films joined from such grains, were grown on polycrystalline or single-crystal Pt substrates by AP-CVD (Methods). A longer growth time was required for graphene grains to form a continuous film. A single-crystal Pt substrate shows similar growth behaviour for graphene as that on polycrystalline Pt. The graphene mentioned in the following discussion was grown on the polycrystalline Pt foils if not specified. The AP-CVD growth conditions avoid the use of specific reaction systems and make the preparation much easier, which will be very useful for the large-scale production of single-crystal graphene at a lower cost. Although the solubility of carbon in Pt is high, ~0.9 at.% at 1,000 °C [26] , we found that monolayer graphene can be easily grown on Pt foils. In contrast to Cu foils [13] , [16] , [19] , Pt foils show a faster growth rate and broader growth windows ( Supplementary Table S1 and Supplementary Fig. S1 ). The growth temperature can be as low as 750 °C when using CH 4 as the carbon source, and the graphene can completely cover the Pt surface in several seconds when using a high CH 4 concentration even at 950 °C. To grow individual single-crystal graphene grains and control their size and nucleation density, we stop the CVD growth before adjacent grains join together. We found that, with decreasing growth temperature, the graphene nucleation density increases and consequently the grain size decreases. For example, small graphene grains of less than 1 μm are formed at a growth temperature of lower than 800 °C. In our experiments, we used a growth temperature of 1,040 °C to grow large single-crystal graphene grains and the films joined from them. In addition to the growth temperature, the concentration of CH 4 strongly affects the nucleation density and grain size of graphene on the Pt foils ( Supplementary Fig. S1 ). The lower the concentration of CH 4 used, the larger the graphene grain size produced. As the flow-rate ratio of CH 4 /H 2 decreases from 20/400 to 10/700 and 5/700, where the individual numbers are the flow rates in standard cubic centimetre per minute (sccm), the size of the graphene grains increases from 50 to 100 and 500 μm. Moreover, the graphene grains become more and more regular, with straighter edges. Surprisingly, when the flow rate of CH 4 /H 2 is changed to 4/700, we obtain predominant graphene grains of a perfect hexagon shape with very smooth edges and a lateral size of up to 1.3 mm on a polycrystalline Pt foil ( Fig. 1a,b and Supplementary Fig. S2a–c ). These are larger than the 20-μm hexagonal single-crystal graphene grains grown on Cu by AP-CVD [22] and the 400-μm dendritic single-crystal graphene grown on Cu foils by LP-CVD [19] . 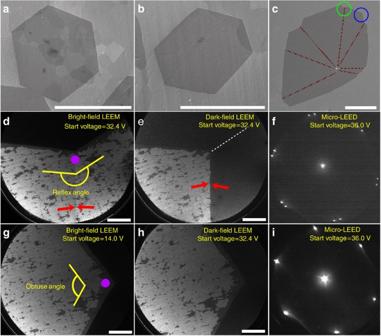Figure 1: Characterization of graphene grains grown on Pt substrates. (a,b) Scanning electron microscope (SEM) images of two hexagonal graphene grains on a polycrystalline Pt foil, which were grown with 4 sccm CH4and 700 sccm H2at 1,040 °C for 180 min. The scale bar in (a) is 1 mm, and in (b) is 0.5 mm. (c) SEM image of an irregular graphene, which contains several grains, on a single-crystal Pt(111). It was grown with 4 sccm CH4and 700 sccm H2at 1,040 °C for 45 min. The red dashed lines indicate the grain boundaries determined by LEEM and micro-LEED patterns. The scale bar is 100 μm. (d,e) Bright-field and dark-field LEEM images recorded at the region with a reflex angle in the green circle in (c). A clear boundary indicated by an arrow was observed in the bright-field LEEM image, and the two sides of this line show sharp contrast in the dark-field LEEM images. The scale bars in (d) and (e) are 10 μm. (f) Micro-LEED pattern taken from the region indicated by a purple dot in (d), showing two spot patterns. (g,h) Bright-field and dark-field LEEM images recorded at the region with an obtuse angle in the blue circle in (c), showing no obvious difference through the whole region, without boundaries being observed. The scale bars in (g) and (h) are 10 μm. (i) Micro-LEED pattern taken from the region indicated by a purple dot in (g), showing only one pattern. For details about the black bubble-like regions in (d–h), seeSupplementary Fig. S5. Figure 1: Characterization of graphene grains grown on Pt substrates. ( a , b ) Scanning electron microscope (SEM) images of two hexagonal graphene grains on a polycrystalline Pt foil, which were grown with 4 sccm CH 4 and 700 sccm H 2 at 1,040 °C for 180 min. The scale bar in ( a ) is 1 mm, and in ( b ) is 0.5 mm. ( c ) SEM image of an irregular graphene, which contains several grains, on a single-crystal Pt(111). It was grown with 4 sccm CH 4 and 700 sccm H 2 at 1,040 °C for 45 min. The red dashed lines indicate the grain boundaries determined by LEEM and micro-LEED patterns. The scale bar is 100 μm. ( d , e ) Bright-field and dark-field LEEM images recorded at the region with a reflex angle in the green circle in ( c ). A clear boundary indicated by an arrow was observed in the bright-field LEEM image, and the two sides of this line show sharp contrast in the dark-field LEEM images. The scale bars in ( d ) and ( e ) are 10 μm. ( f ) Micro-LEED pattern taken from the region indicated by a purple dot in ( d ), showing two spot patterns. ( g , h ) Bright-field and dark-field LEEM images recorded at the region with an obtuse angle in the blue circle in ( c ), showing no obvious difference through the whole region, without boundaries being observed. The scale bars in ( g ) and ( h ) are 10 μm. ( i ) Micro-LEED pattern taken from the region indicated by a purple dot in ( g ), showing only one pattern. For details about the black bubble-like regions in ( d – h ), see Supplementary Fig. S5 . Full size image It is well known that the catalytic decomposition of hydrocarbons on metals, which produces active carbon species, is an important step for the CVD growth of graphene. At the same time, molecular hydrogen in a CVD system for the growth of graphene will dissociate on the metals and form active atomic H, which subsequently etches away weak carbon–carbon bonds [27] . Therefore, the nucleation, growth and grain shape of graphene are strongly affected by competition between these two processes. By decreasing the flow rate of CH 4 , the formation of active carbon species becomes weaker, and this consequently suppresses graphene nucleation. Therefore, the nucleation density of graphene is low at a low CH 4 /H 2 flow-rate ratio leading to the growth of large graphene grains. In some cases, we can even obtain only one single hexagonal grain nucleus over a region of 2.5×2.5 mm ( Supplementary Fig. S3 ). In addition, the armchair and zigzag edges of graphene have different stabilities [22] , [28] . Therefore, the graphene edges become regular and straighter, because edges with a low stability are selectively etched away by an active atomic H when the CH 4 /H 2 flow rate ratio is low. Small bilayer or few-layer regions sometimes were also observed on big graphene grains, as shown in Fig. 1a,b . We suggest that the formation of these structures occurs when the amount of active carbon species produced exceeds what is required for the monolayer graphene growth, such as the beginning of the graphene growth or the different catalytic activities of Pt in different regions. Usually, a temperature higher than 1,000 °C is required for the CVD growth of graphene on Cu, using CH 4 as the carbon source [13] , [14] , [16] , [19] , [20] , [21] , [22] . The fact that graphene can grow on Pt at a relatively low temperature (750 °C) indicates that Pt has a stronger catalytic ability for CH 4 dissociation than Cu, which is consistent with reported theoretical calculations [29] . In contrast to Cu, Pt also has a much stronger catalytic ability for H 2 dissociation to form active atomic H [30] . Note that the CH 4 flow rate (4 sccm) is very low and the H 2 flow rate (700 sccm) is very high for the CVD growth of large single-crystal graphene on Pt, which leads to a low concentration of carbon species and a high concentration of atomic H. We should point out that no graphene was grown on Cu under such conditions, because of the much weaker catalytic ability of Cu for the dissociation of CH 4 . Therefore, we believe that the different catalytic abilities of Pt and Cu for the dissociation of CH 4 and H 2 , the use of a very low CH 4 /H 2 flow rate ratio, and the resultant stronger etching ability for the carbon–carbon bonds is responsible for the much lower nucleation density of graphene on Pt than on Cu, leading to the formation of much larger graphene grains on Pt. Characterizations of single-crystal graphene grains We characterized the large graphene grown on Pt substrates by low-energy electron microscopy (LEEM) and selected-area low-energy electron diffraction (micro-LEED) [18] . Because of the necessity of a smooth Pt substrate required by these techniques, we used single-crystal Pt(111) to grow graphene for characterization. Similar to polycrystalline Pt, many hexagonal graphene grains, as shown in Supplementary Fig. S4 , were formed on Pt(111) at a low CH 4 /H 2 flow rate ratio. Here we analysed an irregular graphene, which has reflex and obtuse angles at its edges, as shown in Fig. 1c . The bright-field LEEM image of the graphene region with a reflex angle shows a clear boundary indicated by an arrow in Fig. 1d , and more importantly, the two sides of this line give a sharp contrast in the corresponding dark-field LEEM image ( Fig. 1e ). The micro-LEED was recorded from a position on this boundary indicated by the purple dot in Fig. 1d . It shows two spot patterns and confirms that the graphene edge with a reflex angle has two different crystal orientations with the line being the grain boundary ( Fig. 1f ). In contrast, the graphene edge with an obtuse angle contains only one crystal orientation, as it shows no contrast difference both in the bright-field and dark-field LEEM images even at various starting voltages. The micro-LEED recorded from the purple dot in Fig. 1g shows only one spot pattern ( Fig. 1i ). A complete survey of this graphene and many other graphene domains gives the same result, that is, the graphene domains with reflex angles have two different crystal orientations, but those with obtuse angles have only one orientation. On the basis of the above observations, we consider that the graphene grain shown in Fig. 1a or b is a single crystal, but the graphene shown in Fig. 1c is a polycrystal and not a single crystal. All the confirmed grain boundaries in this graphene are labelled by red lines in Fig. 1c , and most of them are visible in the scanning electron microscope image, possibly owing to the preferential decoration of the grain boundaries with surface contaminants [21] , [31] ( Supplementary Fig. S6 ). It is interesting to find that this graphene comes from one nucleus, which gives rise to several single-crystal grains with different orientations, similar to the graphene grains grown on Cu foils by LP-CVD [21] . Note that the size of the single-crystal grains in this graphene is at least 150 μm, larger than those grown on Cu foils by AP-CVD (usually about 20 μm) [21] , [22] , but little smaller than the dendritic graphene grown on Cu by LP-CVD [19] . It is first important to note that the predominant hexagonal graphene grains grown on Pt substrates have no reflex angle at the edges and no visible lines in their planes even in high-resolution scanning electron microscope images. Second, the size of the graphene grains is inversely proportional to the nucleation density of graphene. The nucleation density of graphene grains on Pt at a low CH 4 concentration is very low, with a spacing of more than 1 mm, which provides space for the growth of large graphene grains. Third, with increasing growth time, no new nuclei are observed and only the continuous growth of graphene grains is observed. The lateral size of the graphene grains is roughly proportional to the growth time, with a mean growth rate of ~4 μm min −1 under the present growth conditions, which is about four times faster than that (~1 μm min −1 ) of the growth of hexagonal graphene grains on Cu. All the above facts indicate that the hexagonal grains with obtuse angles grown on Pt substrates should be single-crystal graphene grains, which are similar to the hexagonal single-crystal graphene grains grown on Cu foils by AP-CVD [22] , but have a much larger size up to more than a millimetre. It is worth noting that, by further increasing the growth time, large graphene grains join together and eventually form a continuous graphene film with grain boundaries, shown in Fig. 2 . 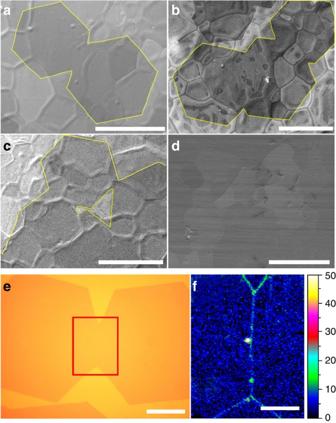Figure 2: Coalescence of graphene grains. Scanning electron microscope (SEM) image of the coalescence of different graphene grains: (a) two; (b) three; (c) many; (d) continuous graphene film formed from grains. The graphene film completely covers the Pt substrates without any gaps. (e) Optical image of two coalesced graphene grains. (f) Raman mapping of the intensity of D band (1,300–1,400 cm−1) at the joint area of the two coalesced grains indicated by a red box in (e). The strong intensities along the line in the mapping indicate a grain boundary. The scale bars in (a–d) are 400 μm, in (e) 50 μm, and in (f) 20 μm. Figure 2: Coalescence of graphene grains. Scanning electron microscope (SEM) image of the coalescence of different graphene grains: ( a ) two; ( b ) three; ( c ) many; ( d ) continuous graphene film formed from grains. The graphene film completely covers the Pt substrates without any gaps. ( e ) Optical image of two coalesced graphene grains. ( f ) Raman mapping of the intensity of D band (1,300–1,400 cm −1 ) at the joint area of the two coalesced grains indicated by a red box in ( e ). The strong intensities along the line in the mapping indicate a grain boundary. The scale bars in ( a – d ) are 400 μm, in ( e ) 50 μm, and in ( f ) 20 μm. Full size image Nondestructive transfer of graphene from Pt substrates The currently used etching-based transfer methods are not suitable for the transfer of graphene grown on Pt, as Pt is chemically inert and more expensive compared with Cu and Ni. Recently, an electrochemical delamination method was reported to transfer graphene grown on Cu [25] , but it was found that a thin layer of Cu, about 40 nm thick, was etched away during one transfer process. For graphene grown on Pt substrates, we have developed a bubbling transfer process, similar to the recently reported method [25] , to transfer the material based on a water electrolysis process [32] ( Fig. 3 ). After CVD growth, a Pt substrate with the graphene grown on it was first spin-coated with polymethyl methacrylate (PMMA) followed by curing. Then the PMMA/graphene/Pt was dipped into an NaOH aqueous solution and used as the cathode of an electrolysis cell with a constant current supply. It is worth noting that the graphene would be easily oxidized if the PMMA/graphene/Pt was used as the anode. At the negatively charged cathode, a water reduction reaction took place to produce H 2 . The reaction can be represented as follows: We observed that the PMMA/graphene layer was detached from the Pt substrate after tens of seconds as a result of the formation of a large number of H 2 bubbles at the interface between the graphene and Pt substrate. This is much faster than the detachment of graphene by substrate etching, which usually takes tens of minutes to etch away substrates such as Cu and Ni. After cleaning with pure water, the floating PMMA/graphene layer was stamped at the target substrate. Finally, the PMMA was removed by acetone, and the graphene grains or films were transferred to the substrate successfully. 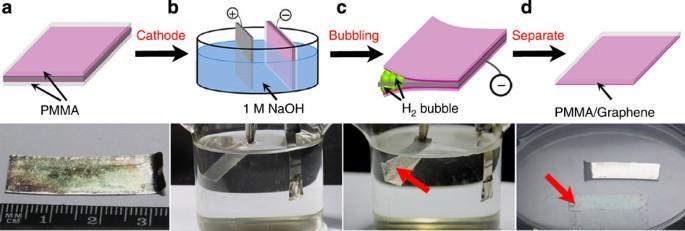Figure 3: Illustration of the bubbling transfer process of graphene from a Pt substrate. (a) A Pt foil with grown graphene covered by a PMMA layer. (b) The PMMA/graphene/Pt in (a) was used as a cathode, and a Pt foil was used as an anode. (c) The PMMA/graphene was gradually separated from the Pt substrate driven by the H2bubbles produced at the cathode after applying a constant current. (d) The completely separated PMMA/graphene layer and Pt foil after bubbling for tens of seconds. The PMMA/graphene layer is indicated by a red arrow in (c) and (d). Figure 3: Illustration of the bubbling transfer process of graphene from a Pt substrate. ( a ) A Pt foil with grown graphene covered by a PMMA layer. ( b ) The PMMA/graphene/Pt in ( a ) was used as a cathode, and a Pt foil was used as an anode. ( c ) The PMMA/graphene was gradually separated from the Pt substrate driven by the H 2 bubbles produced at the cathode after applying a constant current. ( d ) The completely separated PMMA/graphene layer and Pt foil after bubbling for tens of seconds. The PMMA/graphene layer is indicated by a red arrow in ( c ) and ( d ). Full size image Notably, the Pt substrate is chemically inert to the electrolyte and is not involved in any chemical reactions during this transfer process. Therefore, the bubbling delamination method does not destroy the Pt substrate and allows for repeated use of the Pt for the CVD growth of graphene without limit. This is completely different from the currently used etching transfer processes [10] , [11] , [12] , [13] , [14] , [15] , [16] , [19] , [20] , [21] , [22] . In addition, the transferred graphene is free of metal residues, which are usually found in the graphene transferred by the etching process [20] . This bubbling method provides a general strategy to transfer graphene grown on chemically inert noble substrates, such as Pt, Ru, Ir, and so on. We experimentally proved that it can also be used to transfer graphene grown on Cu or Ni onto other substrates. Different from chemically inert noble substrates, however, Cu and Ni were easily oxidized and slightly dissolved during the bubbling transfer process, because of their high chemical reactivity with electrolyte. Therefore, the transfer for graphene on Cu and Ni is intrinsically a partial substrate-etching process instead of a totally non-destructive process. This observation is consistent with recent reported result [25] . 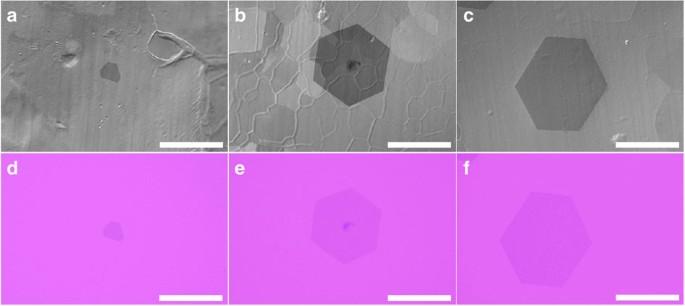Figure 4: Hexagonal graphene grains grown on Pt foils and transferred to Si/SiO2substrates. (a–c) Scanning electron microscope (SEM) images of hexagonal graphene grains grown on Pt foils with different growth times of 60 (a), 120 (b) and 180 min (c), showing that their sizes are roughly proportional to the growth time. The reaction temperature was 1,040 °C, and the flow rates of CH4and H2were 4 and 700 sccm, respectively. (d–f) Optical images of the graphene grains in (a–c) transferred to Si/SiO2substrates by the bubbling transfer process, showing that the transferred graphene grains perfectly retain their original shapes. The scale bars in (a–f) are 400 μm. Figure 4 shows three hexagonal graphene grains grown on polycrystalline Pt foils with different growth times ( Fig. 4a–c ) and the corresponding optical images of those transferred onto Si/SiO 2 substrates with 280 nm thick oxide layer ( Fig. 4d–f ) by the bubbling transfer method. It is important to note that the transferred graphene grains perfectly preserve their original shapes. We found that the transferred graphene films show uniformity over a large area and completely preserve the shape of the Pt substrates used for growth without any cracks ( Fig. 5a,b ). These results indicate that this bubbling transfer process is nondestructive to graphene. A rough analysis of the optical image over a whole graphene film (1×3 cm 2 ) shows that more than 98% of the area is a monolayer graphene (light pink area), with the rest being bilayer and few-layer graphene (dark pink area). The inset in Fig. 5b shows a high-resolution transmission electron microscope image of the monolayer graphene. We also measured the height of more than 900 wrinkles by atomic force microscopy. The wrinkles mostly have a height of less than 2 nm, and the average height fitted by Gaussian distribution is about 0.8 nm ( Fig. 5c ), which is much lower than those of graphene grown on Cu [14] and Ni [33] . The lower wrinkle height is due to the smaller difference in thermal expansion coefficient between Pt and graphene, and should result in lower electron scattering in these graphene. Figure 4: Hexagonal graphene grains grown on Pt foils and transferred to Si/SiO 2 substrates. ( a – c ) Scanning electron microscope (SEM) images of hexagonal graphene grains grown on Pt foils with different growth times of 60 ( a ), 120 ( b ) and 180 min ( c ), showing that their sizes are roughly proportional to the growth time. The reaction temperature was 1,040 °C, and the flow rates of CH 4 and H 2 were 4 and 700 sccm, respectively. ( d – f ) Optical images of the graphene grains in ( a – c ) transferred to Si/SiO 2 substrates by the bubbling transfer process, showing that the transferred graphene grains perfectly retain their original shapes. The scale bars in ( a – f ) are 400 μm. 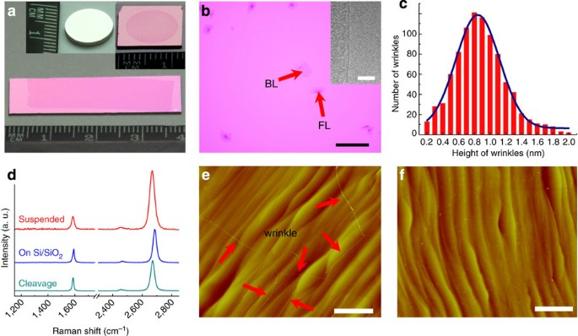Figure 5: Graphene films transferred from Pt substrates. (a) Photograph of a graphene film transferred from a polycrystalline Pt foil to a Si/SiO2substrate. The insets show the as-grown graphene on Pt(111) (left) and transferred to a Si/SiO2substrate (right). (b) Typical optical image of the transferred graphene on a Si/SiO2substrate, showing mostly monolayer with some bilayer (BL) and few-layer (FL) regions. The inset shows a transmission electron microscope image of a monolayer graphene edge. The scale bar is 100 μm. (c) Statistical height distribution of more than 900 wrinkles in the transferred graphene on a Si/SiO2substrate; the average height of the wrinkles is ~0.8 nm. (d) Raman spectra of the monolayer graphene prepared by microcleavage of graphite and those transferred from Pt foils onto Si/SiO2and above a trench in the surface of Si/SiO2. (e,f) Atomic force microscopy images of the Pt(111) surface after graphene growth (e) and after bubbling transfer (f), showing the Pt(111) retains its original structure after transfer. The wrinkles in (e) confirm the existence of graphene. The scale bars in (e) and (f) are 2 μm. Full size image Figure 5: Graphene films transferred from Pt substrates. ( a ) Photograph of a graphene film transferred from a polycrystalline Pt foil to a Si/SiO 2 substrate. The insets show the as-grown graphene on Pt(111) (left) and transferred to a Si/SiO 2 substrate (right). ( b ) Typical optical image of the transferred graphene on a Si/SiO 2 substrate, showing mostly monolayer with some bilayer (BL) and few-layer (FL) regions. The inset shows a transmission electron microscope image of a monolayer graphene edge. The scale bar is 100 μm. ( c ) Statistical height distribution of more than 900 wrinkles in the transferred graphene on a Si/SiO 2 substrate; the average height of the wrinkles is ~0.8 nm. ( d ) Raman spectra of the monolayer graphene prepared by microcleavage of graphite and those transferred from Pt foils onto Si/SiO 2 and above a trench in the surface of Si/SiO 2 . ( e , f ) Atomic force microscopy images of the Pt(111) surface after graphene growth ( e ) and after bubbling transfer ( f ), showing the Pt(111) retains its original structure after transfer. The wrinkles in ( e ) confirm the existence of graphene. The scale bars in ( e ) and ( f ) are 2 μm. Full size image To determine the quality of the graphene obtained, we performed Raman measurements on the graphene transferred to Si/SiO 2 and above a trench on the surface of Si/SiO 2 (suspended graphene). Both samples show no obvious D band ( Fig. 5d ). The intensity ratio of D band to G band ( I D / I G ) is less than 5%, with most being smaller than 2% ( Supplementary Fig. S7 ). This result reveals that the graphene is almost defect-free. The full width at half-maximum (FWHM) of the 2D band of graphene on Si/SiO 2 is in the range of 20–35 cm −1 , with most being ~25 cm −1 ( Supplementary Fig. S7 ). This value is comparable to, or narrower than, those of CVD-grown graphene films and single-crystal graphene on Cu [19] , and comparable to those of microcleavage graphene from graphite [34] . The graphene film on the Si/SiO 2 substrate also shows typical features of p-doping [35] . First, the G and 2D bands upshift to ~1,590 and ~2,685 cm −1 . Second, the G band has a relatively small FWHM, with most being smaller than 18 cm −1 and some being around 10 cm −1 . Third, the intensity ratio of the 2D band to the G band ( I 2D / I G ) is in the range of 2–3. In contrast, the suspended graphene shows a G band at ~1,582 cm −1 , a 2D band at ~2,665 cm −1 , a much broader FWHM of the G band of ~20 cm −1 , and a larger I 2D / I G of ~5 ( Fig. 5d ). These results indicate that the graphene grown on polycrystalline Pt and transferred by the bubbling method intrinsically should have a low doping level. The doping of graphene on Si/SiO 2 substrates arises from trapped charges in the oxide or at the graphene-oxide interface. The high quality of the graphene also indicates that the electrochemical redox reaction involved in the bubbling transfer process did not introduce defects into the graphene. We have also examined the re-use of the Pt substrates after the CVD growth and bubbling transfer process. To investigate any surface change, we used single-crystal Pt(111) as a growth substrate. The wrinkles on the Pt(111) show the existence of graphene ( Fig. 5e ). It is important to note that atomic terraces are maintained without any degradation of roughness even after hundreds of growth and transfer cycles, and no graphene fragments and wrinkles remain ( Fig. 5f ). These results confirm that the bubbling transfer is nondestructive, not only to the graphene but also to the Pt substrate. Therefore, the Pt substrate can be repeatedly used. Moreover, for the same re-used Pt substrate, no obvious structure changes were observed in the graphene films and graphene grains under the same growth conditions after more than 100 transfers ( Supplementary Figs S2 and S8 ). In fact, the polycrystalline Pt foils and single-crystal Pt(111) used in this study have already been re-used more than 1,000 and 200 times, respectively. This nondestructive bubbling transfer process enables the almost unlimited use of growth substrates, which will reduce environmental pollution caused by conventional etching and the production cost of graphene, and is especially important for the transfer of graphene grown on single crystal or noble metal substrates. To evaluate the electronic quality of the transferred graphene, we fabricated back-gate field-effect transistors on Si/SiO 2 substrates, using Ti/Au (5/40 nm) as the source and drain electrodes with a separation of 10 μm. All the transport characteristics of the device were measured in a probe station under ambient conditions. Along with a device model [36] that combines the minimum carrier density at the Dirac point, the dielectric and the quantum capacitances, the measured data and the fitting result are shown in Fig. 6 . Consistent with Raman measurements, the positive Dirac point indicates that the transferred graphene is p-type-doped. The extracted carrier mobility of electrons and holes for this device is ~7,100 cm 2 V −1 s −1 , with the residual carrier concentration at the Dirac point of n 0 =~2×10 11 cm −2 . This mobility is larger than, or comparable to, those of single-crystal graphene on Si/SiO 2 substrates recently reported in the literature, for example, ~4,000 cm 2 V −1 s −1 for dendritic graphene obtained by room temperature field-effect transistor measurements [19] and <1,000–10,000 cm 2 V −1 s −1 for hexagonal single-crystal graphene obtained by low-temperature Hall measurements [22] . We believe that the carrier mobility of the single-crystal graphene grown on Pt can be further improved by using boron nitride substrates [37] , [38] to reduce the charge impurities trapped in SiO 2 . 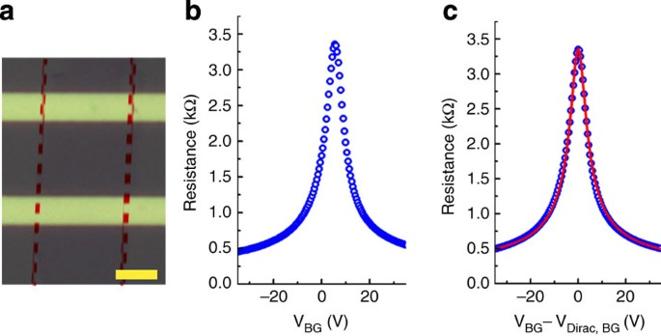Figure 6: Transport property of single-crystal graphene transferred from Pt to a Si/SiO2substrate. (a) Optical image of a back-gate graphene field-effect transistor. The scale bar is 5 μm. (b) Device resistance versus back-gate voltage (VBG) of this graphene field-effect transistor. (c) Device resistance versus VBG−VDirac, BG(VBGat the Dirac point) and with a model fit (solid red line). Figure 6: Transport property of single-crystal graphene transferred from Pt to a Si/SiO 2 substrate. ( a ) Optical image of a back-gate graphene field-effect transistor. The scale bar is 5 μm. ( b ) Device resistance versus back-gate voltage (V BG ) of this graphene field-effect transistor. ( c ) Device resistance versus V BG −V Dirac, BG (V BG at the Dirac point) and with a model fit (solid red line). Full size image CVD growth of graphene on Pt Graphene was grown on 200-μm thick Pt foils (99.9 wt.% metal basis) or Pt(111) (MaTeck, diameter 10 mm×thickness 1 mm, polished <30 nm) under AP-CVD. All the flow rates were measured by mass flow metres calibrated by N 2 in units of sccm. A typical growth procedure is as follows: a piece of Pt foil or Pt(111) was loaded into a fused silica reaction tube, then heated to 1,040 °C with the protection of H 2 (700 sccm); the Pt foil or Pt(111) was annealed at 1,040 °C for 10 min in H 2 to remove possible residual carbon and organic substances; growth was initiated by introducing CH 4 , and maintained for a certain time; the Pt foil or Pt(111) was quickly pulled out of the high-temperature zone, the furnace was shut down, and the CH 4 was turned off when the furnace temperature was lower than 650 °C. The structure and grain size of the graphene strongly depend on the experimental conditions and growth time. Bubbling transfer from Pt substrates For bubbling transfer of graphene, Pt substrates with the grown graphene were spin-coated with PMMA (950 kDa molecular weight, 4 wt.% in ethyl lactate) at 2,000 r.p.m. for 1 min, and cured at 180 °C for 30 min. The bubbling time depends on the size of the graphene and the constant current used. For a graphene film of 1×3 cm 2 , 30-s bubbling is enough to completely separate the PMMA/graphene layer from the Pt foil in a 1 M NaOH aqueous solution under a constant current of 1 A. The current density was usually 0.1–1 A cm −2 , and the corresponding electrolytic voltage was usually 5–15 V. Characterization The Raman spectra of graphene were collected using a 532-nm laser under ambient conditions with a JY HR800, and the laser spot size was ~1 μm. The detailed structures of the graphene grains such as grain size and boundary locations and orientations were characterized by LEEM and micro-LEED (with an area of about 5 μm in diameter) in an Elmitec LEEM system (ultrahigh vacuum of ~1×10 −10 Torr). How to cite this article: Gao, L. B. et al . Repeated growth and bubbling transfer of graphene with millimetre-size single-crystal grains using platinum. Nat. Commun. 3:699 doi: 10.1038/ncomms1702 (2012).